Threshold for sand mobility on Mars calibrated from seasonal variations of sand flux Coupling between surface winds and saltation is a fundamental factor governing geological activity and climate on Mars. Saltation of sand is crucial for both erosion of the surface and dust lifting into the atmosphere. Wind tunnel experiments along with measurements from surface meteorology stations and modelling of wind speeds suggest that winds should only rarely move sand on Mars. However, evidence for currently active dune migration has recently accumulated. Crucially, the frequency of sand-moving events and the implied threshold wind stresses for saltation have remained unknown. Here we present detailed measurements of Nili Patera dune field based on High Resolution Imaging Science Experiment images, demonstrating that sand motion occurs daily throughout much of the year and that the resulting sand flux is strongly seasonal. Analysis of the seasonal sand flux variation suggests an effective threshold for sand motion for application to large-scale model wind fields (1–100 km scale) of τ s =0.01±0.0015 N m −2 . The current landscape and stratigraphic observations of Mars attest to the importance of aeolian processes in shaping the planet and building its sedimentary cover [1] , [2] . Aeolian processes are known to dominate the current Martian climate through the modulation of atmospheric thermal forcing by suspended dust [3] , [4] , [5] , [6] . However, the intensity of wind activity has been judged as significantly lower than on Earth, such that recent evidence for currently active dune migration [7] , [8] , [9] and measurements of Martian sand fluxes comparable to terrestrial values [10] came as a surprise. Prevailing expectations based on wind tunnel experiments, theory for initiation of saltation, atmospheric modelling and limited in situ wind measurements suggested that sand-moving winds should be very rare [11] , [12] , [13] , [14] , [15] , [16] . The apparent contradiction between rare implied saltation and reasonably common dust lifting [17] , [18] remains unresolved but has variously been ascribed to the uncertainties in interparticle cohesion, the role of electrostatics, the role of gustiness and the vertical wind shear and suction in dust devils [18] , [19] . Indeed, a major dust storm occurred during the time period between the acquisitions of the two images analyzed in the preceding Nili Patera High Resolution Imaging Science Experiment (HiRISE) study [10] , [20] , allowing the possibility that anomalously high storm winds accounted for a significant fraction of the measured sand flux. Quantitative interpretation of aeolian features and realistic dynamical modelling of the Martian dust cycle are impeded by the difficulty of transferring to Mars the semi-empirical laws of sand transport established for Earth and estimating the time-integrated effect of high-speed winds based on dynamical simulations. An extra uncertainty for dust emission is the question of whether saltation of sand is the dominant mechanism for dust lifting. Saltation appears to be required, given that sand-sized particles (~100 μm) are significantly easier to mobilize than dust (~1 μm) under most reasonable assumptions regarding the interparticle cohesion of dust (particles >100 μm are also progressively harder to mobilize) [1] , [21] . The key parameter for sand motion is the effective stress threshold for sustained saltation [22] . When applied to wind stress output from an atmospheric model, the threshold determines the fraction of the year over which sand transport is active, the seasonal variation of sand fluxes and hence the annual erosive potential, and the seasonal evolution and magnitude of saltation-induced dust lifting. The latter factor yields a feedback loop in the Martian climate system as the mass of dust lofted modifies the atmospheric and surface thermal forcing (due to absorption/emission and shading, respectively), which in turn significantly modifies the strength of surface wind stresses. The identification of a stress threshold appropriate for use in mesoscale and General Circulation Models (GCM), which have computational grid scales of order 1 to 100 km (O[1–100 km]), is thus a crucial factor in simulating and thus better understanding the ‘steady-state’ Martian dust cycle and the initiation and evolution of dust storms. The lack of viable constraints on the stress threshold in O[1–100 km] scale models creates a vast area of plausible domain space within which the dust cycle might be operating [23] , [24] , much of which ultimately will not be relevant to Mars. We estimate an effective threshold from satellite-based observation of sand activity over an area of about 40 km 2 . Sustained sand flux is observed throughout a Mars Year (MY), with strong seasonal variability. Wind simulations applied to a set of sand transport laws provide a predicted sand flux, which is compared with the measured sand flux. We determine the effective shear stress threshold that allows the predicted sand flux to best reproduce the measured sand flux variations. The threshold, estimated at ~0.01±0.0015 N m −2 , is an effective threshold relevant for mesoscale and general circulation modelling in the O[1–100 km] scale range for which the turbulent characteristic of the wind is not resolved (though in such models the amount of turbulence, and its impact on surface exchange of momentum and mixing within the boundary layer, are typically parametrized in some manner). Seasonal sand flux measurement In this study, we examine a time series of HiRISE images [25] of the Nili Patera dune field (8.8° N, 67.3° E) over the course of a MY to determine the seasonal distribution of sand transport. The barchanoid dune field sits in Nili Patera, a 55 km diameter, ~2 km deep caldera at the top of Syrtis Major, a 1,000 × 1,500 km wide shield volcano lying a maximum of ~6 km above the neighbouring Isidis Planitia basin (Isidis) to the east. The dune field covers an area of ~200 km 2 and is located 500 km west of Isidis ( Fig. 1 ). 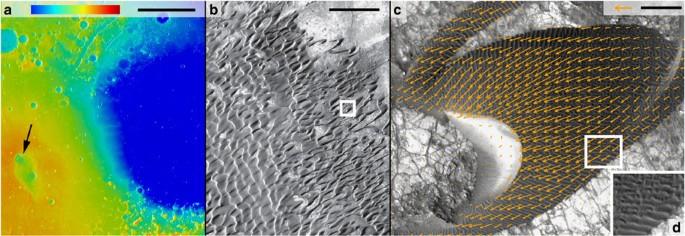Figure 1: Geographic setting and illustration of study area. (a) Location of the Nili Patera dune field (8° N, 67° W) and surrounding topography (Elevation colour scale −4,000 m (blue) to 4,000 m (red); scale bar, 400 km). The arrow points to the Nili Patera caldera that contains the Nili Patera dune field. Notice the large Isidis basin to the east (blue), and smooth topography between the basin rims and Nili Patera. (b) CTX image of the Nili Patera dune front (scale bar, 2 km). The white square indicates the location ofc. (c) HiRISE (ESP_018039_1890) close-up view of a Nili Patera dune with vector field overlay of the ripple migration measured between two time-adjacent HiRISE images (arrow scale 50 cm, scale bar, 50 m). (d) Close-up view (white rectangle inc) of sand ripples. The HiRISE imager aboard the Mars Reconnaissance Orbiter acquired a time series of nine optical images ( Supplementary Table 1 ) at 25 cm pixel scale during MY30 (2010–2011), which cover an area of ~43 km 2 at the eastern (upwind) edge of the dune field. The resolution of the imagery allows observation of ripples that cover the dune surfaces. The sand ripple migration is measured with a precision of a few centimeters from the precise registration and cross-correlation of pairs of successive images using the Co-registration of Optically Sensed Images and Correlation (COSI-Corr) methodology [26] . For each pair of images, a ‘difference’ image is constructed that represents the magnitude of ripple migration during the analyzed time interval. We apply a principal component-based analysis which takes into account the uncertainties assigned to each local measurement, and which produces a time series of ripple migration images with non-correlated noise filtered out (see Methods). We then estimate the average sand flux over each time interval based on ripple migration [6] . The total sand flux, q , scales with the ripple migration sand flux, q r , as q ~ q r 1.2 (ref. 27 ). Our results show a sustained sand flux throughout the year with a strong seasonal variation: during the southern summer period, which includes perihelion (time of closest approach to the Sun), the flux is about three times larger than during the northern summer ( Fig. 2 ). The sand flux measured over a 3-month period in the northern winter of MY28 (2007) (ref. 10 ) is comparable, though about 30% lower, to the winter values obtained for MY30 in this study. We measure only the space- and time-averaged values within each period separating each data acquisition, although a glimpse of the stochasticity of sand-moving winds can be inferred, as follows. All the analyzed pairs show evidence of significant ripple migration, even two pairs of images taken only 17 or 16 days apart (corresponding to the periods with planetocentric solar longitude (Ls)=322–332° and Ls 332–340°, respectively). Over these two consecutive periods the average flux is different by a factor of 2, suggesting that while sand-moving wind events were probably numerous during both of these short-time periods, the variability in frequency, duration and/or strength of these winds must have been large. However, the south-westward direction of the flux, indicated by the migration direction of the sand ripples, is stable over the year ( Supplementary Table 1 ), indicating a fairly constant direction of sand-moving winds. Figure 1: Geographic setting and illustration of study area. ( a ) Location of the Nili Patera dune field (8° N, 67° W) and surrounding topography (Elevation colour scale −4,000 m (blue) to 4,000 m (red); scale bar, 400 km). The arrow points to the Nili Patera caldera that contains the Nili Patera dune field. Notice the large Isidis basin to the east (blue), and smooth topography between the basin rims and Nili Patera. ( b ) CTX image of the Nili Patera dune front (scale bar, 2 km). The white square indicates the location of c . ( c ) HiRISE (ESP_018039_1890) close-up view of a Nili Patera dune with vector field overlay of the ripple migration measured between two time-adjacent HiRISE images (arrow scale 50 cm, scale bar, 50 m). ( d ) Close-up view (white rectangle in c ) of sand ripples. 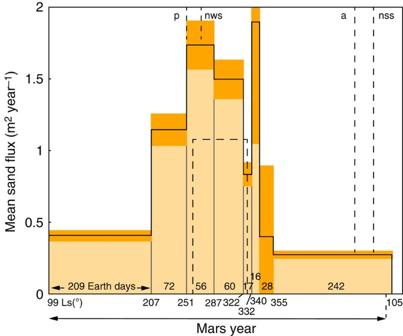Figure 2: Mean sand flux over Nili Patera as a function of solar longitude. The sand flux is derived from measuring ripples migration from the correlation of HiRISE images in MY30 (2010–2011) using COSI-Corr (see Methods). We estimate a mean sand flux for each period separating the dates of acquisition of two successive images (acquisition date is given in solar longitude (Ls) along thex-axis). 1−σerrors of the flux mainly due to acquisition geometric artifact are displayed in dark orange. The sustained sand flux throughout the year, and the significant values obtained over periods of only 16–17 days, suggest that sand-moving winds probably occur daily. The flux is about three times larger in northern winter than in northern summer. The dashed histogram represents the mean sand flux, averaged over the same area, measured in MY28 (2007) (ref.10). The flux in MY28 is smaller than in MY30, probably due to the effect of the large global dust storm, which occurred this year between the two acquisition times. The increased atmosphere opacity would have reduced the effect of Isidis basin on slope flow, resulting in weaker diurnal winds at Nili Patera. The dashed vertical lines indicates the perihelion (p), the northern winter solstice (nws), the aphelion (a) and the northern summer solstice (nss). Full size image Figure 2: Mean sand flux over Nili Patera as a function of solar longitude. The sand flux is derived from measuring ripples migration from the correlation of HiRISE images in MY30 (2010–2011) using COSI-Corr (see Methods). We estimate a mean sand flux for each period separating the dates of acquisition of two successive images (acquisition date is given in solar longitude (Ls) along the x -axis). 1− σ errors of the flux mainly due to acquisition geometric artifact are displayed in dark orange. The sustained sand flux throughout the year, and the significant values obtained over periods of only 16–17 days, suggest that sand-moving winds probably occur daily. The flux is about three times larger in northern winter than in northern summer. The dashed histogram represents the mean sand flux, averaged over the same area, measured in MY28 (2007) (ref. 10 ). The flux in MY28 is smaller than in MY30, probably due to the effect of the large global dust storm, which occurred this year between the two acquisition times. The increased atmosphere opacity would have reduced the effect of Isidis basin on slope flow, resulting in weaker diurnal winds at Nili Patera. The dashed vertical lines indicates the perihelion (p), the northern winter solstice (nws), the aphelion (a) and the northern summer solstice (nss). Full size image Atmospheric models on various scales show that the circulation at Nili Patera is dominated by a combination of the tropical-mean overturning (‘Hadley’) circulation, thermal tides and slope flows associated with the dichotomy boundary and the Isidis basin [28] , [29] , [30] , [31] . Nili Patera is located roughly 9° N of the equator within the seasonally reversing Hadley circulation. During northern summer, the intertropical convergence zone (the location of mean upwelling in the Hadley circulation) is displaced northward of Nili Patera. The cross-equatorial surface expression of this cell (the ‘monsoonal’ circulation) curves due to planetary rotation, yielding mean north-eastward winds at the latitude of Nili Patera. This flow reverses in southern summer, generating south-westward winds. A significant thermal tide [5] is superposed on the monsoonal flow, yielding major daily variations of wind speed and direction, with the latter rotating over a full cycle during the day. Finally, the daily solar heating of the surface in the presence of the dichotomy boundary and the Isidis impact basin yields strong daytime winds that blow up the rim of the basin and then flow radially outward for hundreds of kilometers, contributing west-south-westward winds to the circulation at Nili Patera ( Fig. 1 ). By contrast, nighttime winds that flow down the Isidis rim do not significantly influence Nili Patera flows. We observe that ripple migration occurs throughout the year, and remarkably keeps a south-westward direction, suggesting that sand-moving winds are most likely dominated by the daily flows running outward over the southern highlands from the Isidis basin rim. The peak speed of these winds varies over the year due to the variation of solar heating of the surface with season that is produced for Mars’s current orbital configuration (specifically its obliquity and eccentricity). In southern summer the background winds of the Hadley circulation also blow towards the south-west, reinforcing the Isidis basin topographic forcing. The lower sand flux in MY28 compared with MY30 at the same time of year ( Fig. 2 ) additionally suggests that the global dust storm of MY28 may have inhibited sand transport. Observations from the Martian surface during the 1977a and b dust storms show that increased atmospheric opacity during storms reduces the solar heating of the surface. The MY28 storm is thus likely to have damped buoyancy-slope winds at Isidis in that year. Wind shear stress threshold constrain We use the observed seasonal evolution of the sand flux to estimate an effective wind stress threshold. To do so, we simulate the seasonal evolution of sand flux using a numerical atmospheric model, and adjust the stress threshold used in the sand flux equation such that the predicted seasonal flux variation matches the observed one. The physical validity of the model wind fields are tested to some degree via the demand that—for some choice of threshold—they fit the evolution of the sand flux throughout the year. Our numerical modelling of the wind field uses the MarsWeather Research and Forecast (WRF) system [30] , [32] , a multiscale, nonhydrostatic Mars atmospheric model based on the NCAR WRF system [33] . The model was sampled in seasonal windows over the annual cycle, with near-surface winds, densities and wind stresses output every Martian minute (1/1440th of a Martian day or sol; also see Methods) on a grid spacing scale of 120 km (O[120 km]). We also ran a mesoscale model on a scale of O[1.5 km], not continuously through the year because of the massive computing time that would involve, but for periods of ~5–10 continuous days, every 30° Ls. We find that the two models yield similar output ( Supplementary Fig. 1 ), which suggests that the winds captured by the O[120 km] simulation dominate even in the presence of more local flows. We therefore infer that—whereas the seasonal variation of sand flux predicted by the model is very sensitive to the choice of wind stress threshold—the stress threshold for scales O[1–100 km] should be consistent with the one defined from the O[120 km] scale; we assume so for the rest of the study. A variety of sand transport laws have been proposed which relate the sand flux to the wind stress, τ , in excess of some threshold wind stress, τ s , which is the minimal threshold shear stress required to sustain transport, once initiated. Most agree that sand flux scales between the square and the cube of the frictional velocity . To investigate the sensitivity of our analysis to the chosen law, we predict the sand flux, q , using six different equations (see Methods). 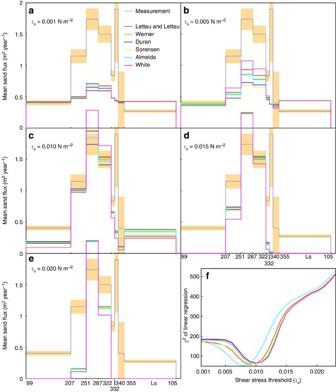Figure 3: Comparison of measured and predicted sand fluxes computed for different shear stress threshold. Shear stress thresholds (τs) from 0.001 to 0.024 N m−2with a step of 0.001 N m−2were tested. Only five of these tests are represented here (a–e). The grey histogram and orange bars respectively represent the measured sand flux and its 1−σerror; the coloured histograms represent the predicted sand fluxes computed from GCM wind output and six transport laws: equation 1 (red); equation 2 (green); equation 3 (blue); equation 4 (yellow, using α=0, β=3.0, γ=2.1 as proposed for a grain size of 170 μm22), equation 5 (cyan), equation 6 (magenta). Equation 4 has been also tested for grain size of 125, 242, and 320 μm, with obtained threshold within 5.10−5N m−2of the threshold for grain size 170 μm. The coloured plots are linearly scaled according to the linear regression between the predicted and measured fluxes. (f) displays theχ2of the linear regression for the set of threshold and transport laws tested. The best linear correlation minimum is obtained for a shear stress threshold between 0.008 and 0.01 N m−2depending on the transport law considered, indicating a weak sensitivity of the stress threshold to the transport law considered. Figure 3 shows the seasonal evolution of sand flux predicted at O[120 km] for the 6 sand flux formulations, and for 5 of the 25 values of the stress threshold examined in this study. The most noticeable aspects of these results are the similarity of the predicted sediment fluxes between the six transport laws tested, and that a strong seasonal variation is predicted in all cases. However, the observed ratio of the summer to winter sand flux is globally reproduced in the predictions for only a limited range of threshold stresses. If the threshold is >0.015 N m −2 , the predicted summer flux drops to nearly zero and the predicted ratio of winter to summer sand flux is significantly too large. Conversely, if the stress threshold is <0.05 N m −2 , the predicted ratio of winter to summer sand flux is too small, less than half the ratio observed. The correlation is generally good, with the exception of the two shortest periods (Ls 322–355° and Ls 355–105°), possibly due to uncertainties in the measurements or to the stochastic nature of the sand-moving winds as discussed above. The effective shear stress threshold for sustained sand motion is thus estimated to be ~ τ s =0.01±0.0015 N m −2 for simulation at a grid scale of O[1–100 km] ( Fig. 4 ). Figure 3: Comparison of measured and predicted sand fluxes computed for different shear stress threshold. Shear stress thresholds ( τ s ) from 0.001 to 0.024 N m −2 with a step of 0.001 N m −2 were tested. Only five of these tests are represented here ( a – e ). The grey histogram and orange bars respectively represent the measured sand flux and its 1− σ error; the coloured histograms represent the predicted sand fluxes computed from GCM wind output and six transport laws: equation 1 (red); equation 2 (green); equation 3 (blue); equation 4 (yellow, using α=0, β=3.0, γ=2.1 as proposed for a grain size of 170 μm [22] ), equation 5 (cyan), equation 6 (magenta). Equation 4 has been also tested for grain size of 125, 242, and 320 μm, with obtained threshold within 5.10 −5 N m −2 of the threshold for grain size 170 μm. The coloured plots are linearly scaled according to the linear regression between the predicted and measured fluxes. ( f ) displays the χ 2 of the linear regression for the set of threshold and transport laws tested. The best linear correlation minimum is obtained for a shear stress threshold between 0.008 and 0.01 N m −2 depending on the transport law considered, indicating a weak sensitivity of the stress threshold to the transport law considered. 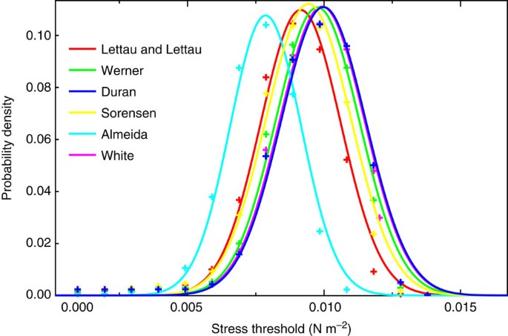Figure 4: Probability density function of the shear stress threshold for various transport laws. The crosses are the Probability Density Function (PDF) at each of the threshold values tested; the continuous curves show best-fitting Gaussian curves. The optimal threshold values and confidence level (at the 1−σconfidence level) are 0.009±0.00149 N m−2, 0.0091±0.00146 N m−2, 0.0098±0.00152 N m−2, 0.01±0.00155 N m−2, 0.0094±0.00155 N m−2, 0.0079±0.00129 N m−2for equation 1 (red), equation 2 (green), equation 3 (blue), equation 4 (yellow), equation 5 (cyan) and equation 6 (magenta), respectively. To account for all the un-modelled sources of error from the measurement, transport law and atmospheric simulations, the sand flux measurements errors were scaled such that the reducedχ2of the linear regression falls to unity. Full size image Figure 4: Probability density function of the shear stress threshold for various transport laws. The crosses are the Probability Density Function (PDF) at each of the threshold values tested; the continuous curves show best-fitting Gaussian curves. The optimal threshold values and confidence level (at the 1− σ confidence level) are 0.009±0.00149 N m −2 , 0.0091±0.00146 N m −2 , 0.0098±0.00152 N m −2 , 0.01±0.00155 N m −2 , 0.0094±0.00155 N m −2 , 0.0079±0.00129 N m −2 for equation 1 (red), equation 2 (green), equation 3 (blue), equation 4 (yellow), equation 5 (cyan) and equation 6 (magenta), respectively. To account for all the un-modelled sources of error from the measurement, transport law and atmospheric simulations, the sand flux measurements errors were scaled such that the reduced χ 2 of the linear regression falls to unity. Full size image We note that the effective threshold value is in between the impact thresholds determined from simulations, 0.003 N m −2 (ref. 21 ) and 0.02 N m −2 (ref. 34 ), and much below the fluid threshold estimated at about 0.08 N m −2 (ref. 35 ). However, the significance of this similarity is unclear as the impact thresholds are defined from high resolution turbulence-resolving models, whereas the effective threshold in this study is defined from non-resolving turbulence large-scale simulations. The value of stress threshold inferred should be interpreted as the effective threshold, which is a unique threshold for initiation and sustenance of sand flux, for the instantaneous mean wind over scales from kilometers to a few degrees. This threshold is much lower than would be expected for turbulence-resolving models, wind tunnel experiments or lander-based local in situ observations [1] , [20] . Large-scale models do not resolve boundary layer turbulence (on scales O[1–1,000 m]) and hence do not simulate gust distributions superposed upon the area–mean winds. However, the estimation of the area average of the unresolved eddy wind stresses (the coherent net effect of ‘gustiness’) is a critical component of the surface layer parameterization included within global and mesoscale models, as realistic surface sources and sinks of angular momentum are needed to generate the observed large-scale circulation. Since turbulent gusts represent a distribution about the mean wind speed, there is a monotonic relationship between the area–mean wind stress threshold and the local instantaneous value. Further, the consistency over the Nili dune field over an area O[100 km 2 ] and the barchanoid nature of the dunes suggest that the dunes form under strong mean winds and that the dune field is not dominated by the structure of the O[1–1,000 m] wind field. As such, the stress threshold estimated from the Nili observations is inherently the O[1–100 km] threshold that would result in a distribution of wind stresses such that some fraction of this distribution is above the local stress threshold for grain motion. This study does not address the nature of the mapping from O[1–100 km] scales to the local scale (O[1–1,000 m]), and it should be noted that this mapping may vary spatially with factors such as the interparticle cohesion, grain size or surface roughness. However, the estimation of the O[1–100 km] threshold stresses estimated here is relevant to estimate dust lifting, sand motion, dune formation and aeolian erosion-based global and mesoscale models. Image processing All images were provided by the US Geological Survey (USGS) in a radiometrically calibrated format named ‘balance cube’ (‘balance cube’ are pre-processed Exposure Data Recognizer (EDR) images which can be obtained from HiRISE PIs; alternatively, users can generate ‘balance cube’ equivalent from EDR images using ISIS). Each image came in the form of 9–10 stripes corresponding to each of the charge-coupled device (CCD) array in the broadband ‘red’ channel. The stripes were processed using the USGS recommended procedure with ISIS. The process stitches back the CCD stripes while accounting for any geometric distortions to provide a reconstructed, distortion-free, full image. Camera and orbital geometries were extracted from the SPICE kernels and imported into COSI-Corr along with the images. In addition to the nine images, a stereoscopic pair was acquired at the beginning of the time series to extract a 1 m post-spacing Digital Elevation Model (DEM) of the dune field. The second image of the stereoscopic pair is the first image of the time series. The topography was extracted using BAE SOCET-SET software. Using COSI-Corr, all the images were registered to the first image of the time series, which warrants a perfect registration of the first image to the DEM by construction. Approximately 25 tie-points were selected between the first image and each image of the time series. The tie-points were the same for all images, except where footprint differences prevented it, in which case the tie-points were relocated inside the overlap of the two images. All the tie-points were located on the bedrock, away from the dunes. The tie-points accuracy was optimized with COSI-Corr using a 256 × 256 pixels window size. The average mis-registration at the tie-point locations of the resulting registered pair of images are on the order of a few millimeters, with a s.d. of ~25 cm ( Supplementary Table 1 ). Most of the registration residual comes from unrecorded jitter of Mars Reconnaissance Orbiter during image acquisition and residual in the CCD arrays relative orientations. Images were then orthorectified with COSI-Corr on the same 25 cm resolution grid, using the optimized set of tie-points, the DEM and the ancillary data. Pairs of time-adjacent images were correlated with COSI-Corr using a sliding window of 70 × 70 pixels (17.5 × 17.5 m) and a step of 16 pixels (4 m). Bias in ripple migration maps due to DEM error DEM extraction using a stereoscopic pair of images relies on feature tracking and measurement of feature shift due to the parallax. An underlying assumption to reconstruct a DEM is the stability of the scene between the images’ acquisitions. Indeed, to recover an accurate topography model, parallax is ideally due to topography only, and not to the topography augmented with a physical shift of the terrain. In this study, the DEM extraction on dunes tracks the ripples features to estimate the dune height. Ripples migration between the acquisitions, if any, will therefore bias the overall dune height. To estimate the bias on the ultimate ripple migration maps due to a potentially biased DEM, we estimated the error in elevation, assuming a ripple migration based on the first measurement map. Using this estimated DEM error, we estimated its contribution on all the migration maps by taking into account the stereoscopic angle between each image pairs of the time series. Ripple migration linearly scales with the elevation of the dune [10] , such that the error in elevation will linearly scale with the dune elevation. We estimate the maximum, average and s.d. of the dune elevation error to be 77 cm, 26 cm and 14 cm, respectively. The DEM error contribution to the subsequent ripple migration maps is listed in Supplementary Table 1 , but overall the error is small, about few centimeters, with a maximum of ~20 cm in the worst case (pair 21652 and 22364 with a stereoscopic angle of 17°). Bias in ripple migration maps due to the use of a unique DEM The DEM was generated at the beginning of the time series. The first image is actually part of the stereo pair that was used to extract the topography. The last image of the time series was acquired 700 days later. In the meantime, dunes migrate, such that using a unique DEM may cause a misalignment of dunes with the images. In Bridges et al. [10] , dune migration speed was estimated to ~1 m per year for the fastest dunes. According to the DEM, the slopes of the dunes’ stoss slopes in the ‘axial’ direction are 4–8°. Assuming a dune displacement of 2 m (in 700 days) and a static morphology and height over this time scale, an error of around 28 cm in elevation would be introduced, which would contribute to a maximum of around 8 cm in ripple migration estimation in the worst case (pair 21,652–22,364 with a stereoscopic angle of 17°). Overall, geometric errors due to (1) stability of the ripple between the stereo-pair acquisition and (2) stability of the dunes during the time series time span, can be neglected in view of the measured ripple displacements which are of the order of few meters. Jitter and CCD-induced mis-registration Unrecorded spacecraft jitter during image acquisition causes distortions in the imagery that are not corrected during the orthorectification. These geometric distortions are recovered in the subsequent correlation maps as erroneous ‘displacements’. As seen in Supplementary Figs 2–3 , geometric distortions (most visible on the bedrock area) can be observed in the cross and along-track directions. The cross-track undulations are a direct effect of the jitter and the along-track stripes are caused by the effect of the jitter on the staggered CCD arrays. Collectively, these jitter and CCD artifact (jitter/CCD artifacts) account for up to 1–2 pixels (25–50 cm), and are the largest source of error in the ripple migration estimation. This source of error is accounted for during the weighted linear regression between predicted and measured fluxes (See Methods—Shear stress threshold estimation). Principal component analysis A principal component analysis (PCA) was applied to the time series to filter out measurement noise and to extract the main signal from the data. In practice, we used a weighted low rank approximation of the covariance matrix to account for the missing values (decorrelated pixels), and different noise amplitude between the maps. Noise amplitude between maps can vary due to the irregular time sampling of the acquisitions, which leads to different shadowing effects and temporal changes. We used an adapted version of PCAIM [36] , giving each map a weight inversely proportional to the number of decorrelated points in the data set. The assumption is that a map containing a large number of decorrelated points is a noisier measurement map. Prior to computing the PCA, all displacement maps were time normalized, to account for the unequal time span between pairs. The χ 2 measurement indicates that the first two components of the PCA accounts for 84 and 82% of the time series variance, of the east/west and north/south displacement maps, respectively. Estimates of ripple height The DEM cannot distinguish ripple topography, so we had to assume a standard ripple height. We used the ripple height of 40 cm defined in Bridges et al. [10] In this study, the ripple height was estimated from the HiRISE images, using two approaches:(1) From the ripple wavelength (directly measured on the image) and using the 1:10 ripple height to ripple wavelength ratio commonly found on Earth. (2) From the trace of the ripple footprint on the bedrock (for the ripple on the edges of the dunes) in association with the dune slope (measured from the DEM). Visual observation of the ripple shape shows a stable ripple wavelength in time and space (except at the very base of the dune where ripples nucleate and grow to stable state). This wavelength stability suggests a stable ripple height over time and space as well. Therefore, because ripple height is stationary, and because we are interested in the relative variation of the flux only, the ripple height actual value does not play a role during the linear regression between predicted and measured sand flux. Ripple height would play a definite role if we were to estimate the absolute sand flux quantity however. Sand flux estimation The ripple displacement maps were reconstructed ( Supplementary Figs 4–11 ) using the first two components of the PCA ( Supplementary Figs 2–3 ). The migration azimuth of the ripple is quite stable throughout the year ( Supplementary Table 1 ), and is ~115° from north counterclockwise. This azimuth corresponds also to the azimuth found in Bridges et al. [10] The scattered azimuth distribution for pairs 23,564–23,920 is due to strong un-modelled satellite jitter. To limit the jitter bias in the estimation of the sand flux, the ripple displacements are projected onto the main migration direction, and the average sand flux was estimated for each map using the method described in Bridges et al. [10] Because the displacement maps are co-registered, and because we used the reconstructed maps, the exact same pixels, in location and amount, were used to compute the average reptation sand flux of each displacement map of the time series. Note that the sand flux estimated on every point on the dune scales linearly with the height of the dune [10] , that is, for a given dune, sand flux will vary from approximately no sand flux (base) to a maximum (crest). The average flux computed in this study differs from the traditional ways of quantifying sand flux, for example, at the crest, area based, but is relevant for the temporal evolution analysis. GCM and mesoscale simulations The MarsWRF model [30] , [32] was run at 2° global grid spacing, with four levels of interactive nests used to increase the resolution over the Nili Patera region. Each embedded domain contained 120 × 120 grid points, and had a factor of 3 refinement of the grid (that is, produced a threefold increase in resolution), resulting in a grid spacing of ~1.5 km in the innermost nest, centred on the Nili Patera caldera. MarsWRF, as run for this study, used surface boundary conditions from the 1/64th degree MOLA topographic map, 1/2 degree MOLA roughness map and albedo and thermal inertia maps [30] derived from the Mars Global Surveyor Thermal Emission Spectrometer (MGS-TES). The simulation used the two-stream k-distribution radiative transfer model, treating CO 2 and dust radiative heating [37] and the MRFPBL boundary layer scheme. The dust distribution was defined using the Mars Climate Database ‘MGS’ dust scenario. The model includes a full carbon dioxide cycle that produces roughly 30% variation of atmospheric mass over a MY. The cycle is calibrated with respect to the multi-year Viking lander pressure data sets [30] . The GCM 2° output used in this study was taken from the last year of a multi-year run. The output (drag velocity, air density and vector winds near the surface) was sampled every Martian minute (1/1440th of a Mars day or Sol) over the whole year. Mesoscale simulations were not run for the whole year, but were sampled every minute for ~10 Sols over intervals starting at Ls=0° and every 30° of Ls thereafter. Each mesoscale simulation was initialized using output at the required Ls from the global 2° run, and the first three sols were discarded to avoid ‘spin-up’ effects ( Supplementary Fig. 1 ). Shear stress threshold estimation The objective is to adjust the sand shear stress threshold used with the prediction of atmospheric simulations and a transport law, such that the predicted sand flux matches the observed sand flux (from the imagery). Using the GCM prediction of the wind shear, we tested a total of six transport laws to estimate the shear stress threshold for sustained transport, once initiated. Because we are matching the seasonal variation of flux (that is, the relative flux, rather than the absolute magnitude of flux at a given time) the constants at the start of the equations are factored out: where is the threshold velocity calculated from the atmospheric density, ρ , and stress threshold . Note that while the threshold is often stated in terms of the frictional velocity, as the latter is easier to measure, it is the shear stress that is of primary physical importance for the initiation of grain motion. We estimated the optimal shear stress threshold from the χ 2 -analysis of the best fit (linear regression) between predicted and measured fluxes for a range of threshold values. Two main elements taken into account in the weighted linear regression are detailed below: The measured ripple-induced sand flux represents only the reptation sand flux. However, the total sand flux is composed of the reptation and saltation sand fluxes. Andreotti [27] proposed that the reptation flux scales with u * 2 , and that the total flux scales with , which is a relation also proposed by Werner [39] . We therefore assume the repton flux q r to scale with the total flux q as q ~ q r 1.2 for u * above the threshold. This relation was accounted for during the estimation of the shear threshold, as the predicted sand flux from the simulations represents the total sand flux. The larger source of flux measurement error is the jitter/CCD artifact (Methods—Jitter and CCD-induced mis-registration), which we accounted for in the linear regression as follows. For each pair, the error from the jitter/CCD artifact on the estimated sand flux is quantified: the east/west and north/south displacement maps of the bedrock only (that is, no dunes) are projected on the main migration direction (115°). The average and variance of the ‘equivalent’ sand flux is computed. In an artifact free setup, the average and variance of the resulting ‘equivalent’ sand flux should be null. As expected, the average is close to zero as the satellite ancillary parameters are optimized such that the overall co-registration of the ~25 tie-points located on the bedrock is optimal. The variance however is not null ( Supplementary Table 1 ). Although the CCD/Jitter error is not uniformly distributed on the field area, the bedrock and dunes are sufficiently interlaced to consider the sand flux error estimated from the bedrock to correctly represent the sand flux error on the dunes. This error variance was used as a confidence weight on the measurement during the linear regression. Note: the jitter/CCD artifact does not depend on the time span between acquisitions. However, the resulting ‘equivalent’ sand flux does, and the larger the time span, the smaller the error on the measured sand flux. The reduced χ 2 -curves have a minimum ~10, which indicates that some error sources, whether they originate from the measurement, the simulation or the transport law, are not properly accounted for. One source of error is the stochastic nature of wind events that cannot be captured in the simulations, but observed in the measurements with low time span. To account for the error sources that are not captured, we increased the error on the measurement such that the resultant-reduced χ 2 falls to unity. The resulting probability density function gives us a conservative confidence level on the shear stress and are represented in Fig. 4 . List of software used SOCET-Set . Commercial software provided by BAE Systems ( www.baesystems.com ) used for the DEM generation from stereogrammetry. We followed the procedure recommended by the USGS ( http://webgis.wr.usgs.gov/pigwad/tutorials/socet-set/SocetSet4HiRISE.htm ). Along with the DEM, the two orthorectified images from the stereopairs were generated, and one of them was used as the reference to register the time series to the topography. ISIS . Free, open source image processing software developed and provided by the USGS ( http://isis.astrogeology.usgs.gov/ ). This software was used to pre-process the raw HiRISE imagery into a format that can be handled by COSI-Corr. The ISIS processing also extract the metadata of the images (telemetry, camera geometry and satellite jitter) from the NASA SPICE kernels, and store them into an ascii file that can be read by COSI-Corr. COSI-Corr . Free, not open source software provided by Caltech ( http://tectonics.caltech.edu/slip_history/spot_coseis/ ), and used to orthorectify, register and correlate the image time series. The output of COSI-Corr is the ripple displacement maps. The methodology used to process and generate these images is the one described in the User Guide. The HiRISE capability of COSI-Corr, developed by the authors of this study, will be a part of the next COSI-Corr release. PCAIM . Free and open source software provided by Caltech ( http://tectonics.caltech.edu/resources/pcaim/ ). This software was used to compute the PCA on the HiRISE time series. MarsWRF . Free and open source atmospheric simulation software ( http://planetwrf.com/ ), developed and provided by Ashima Research ( http://ashimaresearch.com/ ). The GCM and mesoscale simulations of the wind regime at Nili Patera were computed using MarsWRF with the parameters that are described in Methods—GCM and mesoscale simulations. How to cite this article: Ayoub, F. et al. Threshold for sand mobility on Mars calibrated from seasonal variations of sand flux. Nat. Commun. 5:5096 doi: 10.1038/ncomms6096 (2014).